Pericytes resident in postnatal skeletal muscle differentiate into muscle fibres and generate satellite cells Skeletal muscle fibres form by fusion of mesoderm progenitors called myoblasts. After birth, muscle fibres do not increase in number but continue to grow in size because of fusion of satellite cells, the postnatal myogenic cells, responsible for muscle growth and regeneration. Numerous studies suggest that, on transplantation, non-myogenic cells also may contribute to muscle regeneration. However, there is currently no evidence that such a contribution represents a natural developmental option of these non-myogenic cells, rather than a consequence of experimental manipulation resulting in cell fusion. Here we show that pericytes, transgenically labelled with an inducible Alkaline Phosphatase CreERT2, but not endothelial cells, fuse with developing myofibres and enter the satellite cell compartment during unperturbed postnatal development. This contribution increases significantly during acute injury or in chronically regenerating dystrophic muscle. These data show that pericytes, resident in small vessels of skeletal muscle, contribute to its growth and regeneration during postnatal life. Satellite cells are myogenic stem/progenitor cells of postnatal skeletal muscle and have a prominent role in tissue growth and regeneration. Recent work has demonstrated that, like embryonic myoblasts, most, if not all, satellite cells in the body originate from the Pax3+/Pax7+ cells in the somites and become detectable in their specific niche, underneath the basement membrane of skeletal muscle fibres, from approximately E16.5 in the mouse [1] , [2] , [3] , [4] . However, numerous reports indicate that, on transplantation, cells from tissues other than muscle (for example, bone marrow, brain, adipose tissue and blood vessels) can fuse with regenerating muscle fibres and also contribute to the satellite cell pool [5] , [6] , [7] , [8] . It is therefore important to understand whether contribution to skeletal muscle by non-myogenic progenitors is restricted to artificial conditions created by transplantation, or whether it occurs during unperturbed pre- and post-natal development. To address this question, we used a Cre-loxP lineage tracing strategy to follow the in vivo fate of progenitors associated with the vasculature. Recently, we reported that pericytes associated with the micro-vasculature of human muscle are able to differentiate into skeletal muscle in vitro and in vivo , on transplantation into dystrophic, immune-deficient mice [9] . A major problem in pericyte biology is the lack of specific markers [10] . Thus, we chose alkaline phosphatase (AP) that, in contrast to other pericyte markers such as the neuro-glial 2 proteoglycan (NG2) [11] or platelet-derived growth factor receptor beta (PDGFRβ) [12] , is not expressed in skeletal muscle fibres, nor in myogenic progenitors, but is restricted to the micro-vasculature of striated muscle in postnatal life. This strategy allowed us to label a subset of pericytes and endothelial cells, as in the mouse both of these cell types express AP. A second reporter mouse Tg:VE-Cadherin ( PAC ) -CreERT2 (ref. 13 allowed us to selectively follow endothelial cell fate inside skeletal muscle. Our data show that during postnatal growth, pericytes, but not endothelial cells, contribute to fibre development and to the satellite cell pool and, that this contribution is further enhanced by acute or chronic tissue regeneration. Alkaline phosphatase is expressed in muscle microvessels In preliminary studies, we examined in great detail the expression of AP in postnatal and adult skeletal muscle. AP expression is robust and widespread in tissues such as intestine, bone and liver, whereas it is restricted to the micro-vasculature of other tissues, such as striated muscles, in many species [14] , [15] , [16] including human [9] . We performed extensive immunofluorescence, confocal analysis on adult and juvenile skeletal muscle to confirm AP expression in vessel-associated cells. Both AP+ endothelial cells and pericytes were unequivocally identified by their anatomical niche and by labelling with different antibodies that recognize either one or the other cell population ( Fig. 1a–l ; Supplementary Fig. S1a–c ). 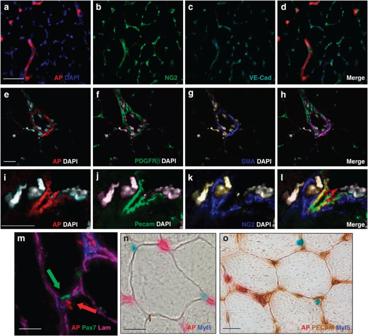Figure 1: AP expression in mouse postnatal skeletal muscle. (a–d) Immunofluorescence analysis on 1-month-old mouse muscle sections shows localization of AP within vessel-associated cells. (a) AP+ cells are stained in red, nuclei are stained in blue by DAPI (b) NG2+ cells are stained in green, (c) Ve-Cadherin+ cells are stained in cyan, (d) merged image. (e–h) AP is expressed by PDGFRβ+/SMA+ pericytes. (e) AP+ cells are stained in red, nuclei are stained in grey by DAPI, (f) PDGFRβ+ cells are stained in green, nuclei are stained in grey by DAPI (g) SMA+ cells are stained in blue and nuclei in grey by DAPI, (h) merged image. (i–l) AP is expressed by Pecam+ endothelial cells, surrounded by an AP-negative pericyte. (i) AP+ cells are stained in red, nuclei are stained in grey by DAPI, (j) Pecam+ cells are stained in green, nuclei are stained in grey by DAPI, (k) NG2+ cells are stained in blue, nuclei are stained in grey by DAPI, (l) merged image. (m) ImmunostainedTAmuscle (15-days-old) shows a Pax7+ satellite cell (green arrow), and an AP+ vessel-associated cell (red arrow); Laminin in magenta. We counted 170 AP+/Pax7− cells and 102 AP−/Pax7+ cells inTAmuscle and 438 AP+/Pax7− cells and 138 AP−/Pax7+ cells inSoleusmuscle: no co-localization is detected. (n,o)Myf5nlacZ/+TAmuscle sections stained for X-gal (blue) and AP (red); Pecam is stained brown in (o). (a–d) Scale bar, 100 μm. (e–o) Scale bar, 20 μm. Figure 1: AP expression in mouse postnatal skeletal muscle. ( a – d ) Immunofluorescence analysis on 1-month-old mouse muscle sections shows localization of AP within vessel-associated cells. ( a ) AP+ cells are stained in red, nuclei are stained in blue by DAPI ( b ) NG2+ cells are stained in green, ( c ) Ve-Cadherin+ cells are stained in cyan, ( d ) merged image. ( e – h ) AP is expressed by PDGFRβ+/SMA+ pericytes. ( e ) AP+ cells are stained in red, nuclei are stained in grey by DAPI, ( f ) PDGFRβ+ cells are stained in green, nuclei are stained in grey by DAPI ( g ) SMA+ cells are stained in blue and nuclei in grey by DAPI, ( h ) merged image. ( i – l ) AP is expressed by Pecam+ endothelial cells, surrounded by an AP-negative pericyte. ( i ) AP+ cells are stained in red, nuclei are stained in grey by DAPI, ( j ) Pecam+ cells are stained in green, nuclei are stained in grey by DAPI, ( k ) NG2+ cells are stained in blue, nuclei are stained in grey by DAPI, ( l ) merged image. ( m ) Immunostained TA muscle (15-days-old) shows a Pax7+ satellite cell (green arrow), and an AP+ vessel-associated cell (red arrow); Laminin in magenta. We counted 170 AP+/Pax7− cells and 102 AP−/Pax7+ cells in TA muscle and 438 AP+/Pax7− cells and 138 AP−/Pax7+ cells in Soleus muscle: no co-localization is detected. ( n , o ) Myf5 nlacZ/+ TA muscle sections stained for X-gal (blue) and AP (red); Pecam is stained brown in ( o ). ( a – d ) Scale bar, 100 μm. ( e – o ) Scale bar, 20 μm. Full size image We never detected AP+ cells that are not associated with small vessels; on the other hand, less than 20% of total vessels express AP. The in vivo expression pattern of AP in postnatal skeletal muscle was also confirmed by analysing mice carrying one copy of the TN-AP β geo allele [17] . In this mouse strain, β-gal+ cells are only associated with vessels, whereas myofibres and satellite cells are always unlabelled ( Supplementary Fig. S1d ). In skeletal muscle, pericytes and satellite cells are often adjacent to each other [18] (arrows in the Fig. 1m ); however, AP was never detected in Pax7+ or MyoD+ satellite cells at any time examined; an example at P7 is shown in Supplementary Figure S1e,f, respectively. These results were confirmed by enzymatic staining for AP on muscles sections from the Myf5 nlacZ/+ mouse (expressing nuclear β-gal only in Myf5+ cells [19] ) ( Fig. 1n ), even after cardiotoxin-induced regeneration ( Supplementary Fig. S1g–j ). Notably, AP activity was invariably detected outside the basement membrane encircling skeletal muscle fibres and co-localized with platelet endothelial cell adhesion molecule (Pecam)-positive vessels ( Fig. 1o ). Moreover, in single myofibres isolated from EDL or Tibialis anterior ( TA ) of P30 Myf5 nlacZ/+ mice, satellite cells were found not to express AP during activation, proliferation or differentiation ( Supplementary Fig. S1k–m ). In contrast, nonpurified primary cultures of skeletal muscle contained both AP+ and Myf5+ cells, but double positive cells were never detected ( Supplementary Fig. S1n ). Satellite cells-derived clones did not express AP during proliferation (5 days in vitro ) or after differentiation (10 days in vitro ) ( Supplementary Fig. S1o,p ). Taken together, these results show that, in mouse postnatal skeletal muscle, AP is only expressed by a subset of vessel-associated cells, whereas myogenic cells and myofibres never express AP. Tissue nonspecific alkaline phosphatase CreERT2 mice Three isoforms of AP have been identified in mouse: the placental (P-AP) and the intestinal (I-AP) isoforms on chromosome 1, and tissue nonspecific AP (TN-AP) on chromosome 4. By RT–PCR with primers specific for the different isoforms [20] , we found that adult skeletal muscle express exclusively TN-AP ( Supplementary Fig. S2a ). To follow the fate of AP+ cells in postnatal skeletal muscle, we generated three transgenic Tg:TN-AP-CreERT2 mouse lines (#3; #6; #12) ( Supplementary Fig. S2b,c ). After crossing with R26R reporter, the three transgenic lines express similar efficiency of Cre recombination, with little variability among different animals. No signal outside AP+ cells was detected in any of the mouse lines. We chose, for the majority of subsequent experiments line #12, whose founder was more fertile. However, several crucial experiments, such as contribution to muscle fibres, were repeated in the different lines, again with similar results. To examine the efficiency of recombination during postnatal skeletal muscle development, we subcutaneously injected Tg:TN-AP-CreERT2:R26R mice with tamoxifen for 3 consecutive days at P6, P7 and P8, and skeletal muscles were analysed 3 days after the last injection. Approximately 70% of AP+ vessels also express β-gal, indicating efficient recombination, and no β-gal+/AP-negative cells were detected ( Fig. 2a ). Whole-muscle X-gal staining revealed β-gal+ vessels as expected (Diaphragm and Quadriceps muscles are shown in Fig. 2b,c , respectively). Moreover we demonstrated, on skeletal muscle sections from Tg:TN-AP-CreERT2 mice that also carry the R26 NZG reporter [21] , that β-gal is expressed by both Pecam+ endothelial cells ( Fig. 2d,e ) and PDGFRβ+ ( Fig. 2f,g ) or NG2+ ( Fig. 2h–k ) pericytes at a ratio of about 1:1 (quantification in Fig. 2l : 500 β-gal+ cells were analysed.). The same results were confirmed also with Tg:TN-AP-CreERT2:R26R mice. ( Supplementary Fig. S2d,e ). After control oil injections no β-gal signal was detected ( Supplementary Fig. S2f,g ). 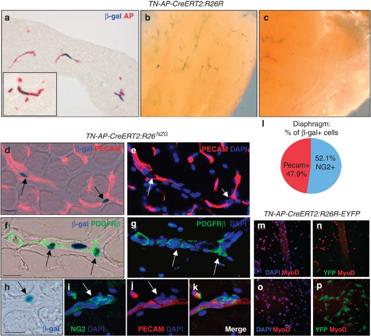Figure 2:Tg:TN-AP-CreERT2mouse generation. (a) Section of Diaphragm muscle from double heterozygousTg:TN-AP-CreERT2:R26Rmice stained for β-gal (blue) and grey (red) 72 h after tamoxifen injection. Double-positive β-gal+/AP+ vessels are clearly visible. High magnification in the inset. Scale bar, 100 μm. (b,c) X-gal whole-mount staining of Diaphragm (b) andQuadriceps(c) fromTg:TN-AP-CreERT2:R26Rmice, 72 h after last tamoxifen injection. (d–k)Tg:TN-AP-CreERT2:R26NZGTricepsmuscle sections, 72 h after tamoxifen injection, stained with X-Gal and antibodies specific for the endothelial or pericyte lineages. (d,e) Two β-gal+/Pecam+ endothelial cells are visible (arrows). Pecam is stained in red, nuclei are counterstained with DAPI. Scale bar, 20 μm. (f,g) Two β-gal+/PDGFRβ+ pericytes surrounding a small vessel. PDGFRβ is stained in green, nuclei are counterstained with DAPI. Scale bar, 20 μm. (h–k) A β-gal+/NG2+ pericyte surrounding a small vessel. Note that the pericyte is negative for the endothelial marker Pecam. NG2 is stained in green; Pecam in red; nuclei are counterstained with DAPI. Scale bar: 20 μm. (l) Distribution of β-gal+ cells within the endothelial and pericyte populations for the Diaphragm muscle; 500 β-gal+ cells were analysed. (m,n) Single fibre preparation fromTg:TN-AP-CreERT2:R26R-EYFP TAmuscle cultured for 5 days with 4-OH tamoxifen and stained with anti-MyoD (red) and anti-GFP antibodies (green); DAPI in blue. No YFP+ cells were found in purified fibre preparations. Scale bars, 50 μm (o,p) Nonpurified cell suspension ofTAmuscle fromTg:TN-AP-CreERT2:R26R-EYFPmice, cultured for 5 days with 4-OH tamoxifen and stained for MyoD (red) and GFP (green); DAPI in blue. Scale bars, 50 μm. Figure 2: Tg:TN-AP-CreERT2 mouse generation. ( a ) Section of Diaphragm muscle from double heterozygous Tg:TN-AP-CreERT2:R26R mice stained for β-gal (blue) and grey (red) 72 h after tamoxifen injection. Double-positive β-gal+/AP+ vessels are clearly visible. High magnification in the inset. Scale bar, 100 μm. ( b , c ) X-gal whole-mount staining of Diaphragm ( b ) and Quadriceps ( c ) from Tg:TN-AP-CreERT2:R26R mice, 72 h after last tamoxifen injection. ( d – k ) Tg:TN-AP-CreERT2:R26 NZG Triceps muscle sections, 72 h after tamoxifen injection, stained with X-Gal and antibodies specific for the endothelial or pericyte lineages. ( d , e ) Two β-gal+/Pecam+ endothelial cells are visible (arrows). Pecam is stained in red, nuclei are counterstained with DAPI. Scale bar, 20 μm. ( f , g ) Two β-gal+/PDGFRβ+ pericytes surrounding a small vessel. PDGFRβ is stained in green, nuclei are counterstained with DAPI. Scale bar, 20 μm. ( h – k ) A β-gal+/NG2+ pericyte surrounding a small vessel. Note that the pericyte is negative for the endothelial marker Pecam. NG2 is stained in green; Pecam in red; nuclei are counterstained with DAPI. Scale bar: 20 μm. ( l ) Distribution of β-gal+ cells within the endothelial and pericyte populations for the Diaphragm muscle; 500 β-gal+ cells were analysed. ( m , n ) Single fibre preparation from Tg:TN-AP-CreERT2:R26R-EYFP TA muscle cultured for 5 days with 4-OH tamoxifen and stained with anti-MyoD (red) and anti-GFP antibodies (green); DAPI in blue. No YFP+ cells were found in purified fibre preparations. Scale bars, 50 μm ( o , p ) Nonpurified cell suspension of TA muscle from Tg:TN-AP-CreERT2:R26R-EYFP mice, cultured for 5 days with 4-OH tamoxifen and stained for MyoD (red) and GFP (green); DAPI in blue. Scale bars, 50 μm. Full size image To further validate this transgenic mouse model and to unequivocally rule out that the Cre recombinase might be activated by satellite cells, we prepared single fibres and nonpurified cells suspension from skeletal muscle of Tg:TN-AP-CreERT2 : R26R-EYFP mice. Both preparations were cultured for 5 days with 4-OH tamoxifen: no yellow fluorescent protein (YFP) positive cells were found in purified, cultured muscle fibres ( Fig. 2m,n ); whereas in nonpurified primary cultures both YFP and MyoD were expressed, but never in the same cell ( Fig. 2o,p ). By RT–PCR, we showed that freshly isolated YFP+ cells from Tg:TN-AP-CreERT2:R26R-EYFP mice (killed 2 days after the last tamoxifen injection), express TN-AP but not Pax7 and Myf5 messenger RNAs, as opposed to freshly isolated SM/C2.6+ satellite cells from the same mice ( Supplementary Fig. S2h ). Moreover, quantitative RT–PCR showed that YFP+ cells express high levels of Cre , while satellite cells isolated from the same mice do not ( Supplementary Fig. S2i ; as positive control, we used C2C12 cells infected with recombinant AAV- Cre ). These results indicate that satellite cells and their derivatives do not express the transgenic TN-AP-CreERT2 construct, both in vivo and in vitro . AP-derived cells contribute to postnatal skeletal muscle To analyse the fate of AP+/β-gal+ cells, Tg:TN-AP-CreERT2:R26R mice were genetically labelled as described above and were killed 8 weeks later, at the end of their growth period. We detected several areas with β-gal+ fibres in all muscles analysed ( Quadriceps , Gastrocnemius and Biceps femoris muscles are shown in Fig. 3a–c ). Skeletal muscle sections showed many β-gal+ muscle fibres together with β-gal+ vessels ( Fig. 3d,e ) and several β-gal+/MyHC+ fibres ( Fig. 3f ). β-gal expression was randomly distributed between fast and slow fibres. The highest percentage of β-gal+ myofibres (7.3±1.2%) was observed in the Diaphragm whereas the lowest was in the TA muscle (0.6±0.2%) ( Fig. 3g ). We also confirmed these results by assaying β-gal activity in homogenates from different muscles (Methods) ( Fig. 3h ). Similar results were obtained using Tg:TN-AP-CreERT2:R26 NZG mice ( Fig. 3i , quantification in Fig. 3g ), where we could clearly detect blue nuclei inside skeletal muscle fibres ( Fig. 3j,k ), ruling out the possibility of nonspecific staining due to β-gal diffusion inside the tissue. Tamoxifen injections at P1, P2 and P3 resulted in high pup lethality and did not significantly increase the percentage of labelled myofibres, suggesting that the contribution of AP-expressing cells to skeletal muscle remains constant in the first week of postnatal life. On the other hand, later tamoxifen injections, from P8 to 1 month of age, resulted in a progressively lower amount of β-gal+ fibres in adult life, indicating that the myogenic potential of AP+ cells decreases with subsequent mouse growth. 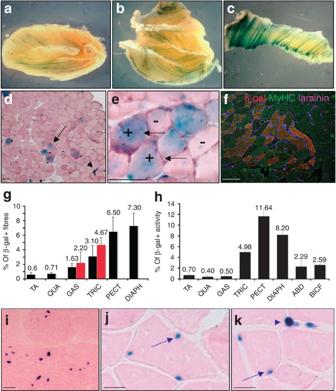Figure 3: Cells derived from TN-AP+ pool contribute to skeletal muscle fibre development. (a–c) β-gal staining of three different muscles, 2 months after tamoxifen injection:Quadriceps(a)Gastrocnemius(b),Biceps femoris(c). (d,e)Quadricepsmuscle sections stained for β-gal; blue fibres (arrow) along with blue vessels (arrowhead) are visible. The sign (+) marks β-gal+ fibres, whereas the sign (−) marks fibres with very low or no β-gal expression. (f) Immunofluorescence on sections from the same muscles shown in (d) and in (e) stained with anti-β-gal (red), anti-MyHC (green) and anti-Laminin (magenta) antibodies confirms the presence of β-gal positive fibres. Scale bar, 100 μm. (g) Quantification of β-gal+ fibres counted on the total fibre number. Different muscles were analysed. Number of experimental animals:n=15 for Tg:TN-AP-CreERT2:R26Rmice, black bars;n=5 forTg:TN-AP-CreERT2:R26NZG, red bars. Error bars represent standard deviation. (h) β-gal activity measurement on muscle homogenates. Standard curve was obtained by different dilutions ofCMV-Cre-R26and wt muscles. β-gal activity obtained 1 week after the last tamoxifen injection inTN-AP-CreERT2:R26Rmice (representing labelling of the vessels) was subtracted from the obtained values. QUA,Quadriceps; GAS,Gastrocnemius; TRIC,Triceps; PECT,Pectoralis; DIAPH, Diaphragm; ABD,Abdominal; BICF,Biceps femoris. Number of experimental animals:n=5. Error bars represent standard deviation. (i–k) Muscle sections ofTg:TN-AP-CreERT2:R26NZGinjected with tamoxifen at P6–P8 and killed 2 months later, stained with X-gal and Eosin. Arrows show β-gal+ nuclei inside skeletal muscle fibres; arrowhead shows β-gal+ nuclei of vessel-associated cells. Scale bar, 100 μm (i) or 20 μm (j,k). Figure 3: Cells derived from TN-AP+ pool contribute to skeletal muscle fibre development. ( a – c ) β-gal staining of three different muscles, 2 months after tamoxifen injection: Quadriceps ( a ) Gastrocnemius ( b ), Biceps femoris ( c ). ( d , e ) Quadriceps muscle sections stained for β-gal; blue fibres (arrow) along with blue vessels (arrowhead) are visible. The sign (+) marks β-gal+ fibres, whereas the sign (−) marks fibres with very low or no β-gal expression. ( f ) Immunofluorescence on sections from the same muscles shown in ( d ) and in ( e ) stained with anti-β-gal (red), anti-MyHC (green) and anti-Laminin (magenta) antibodies confirms the presence of β-gal positive fibres. Scale bar, 100 μm. ( g ) Quantification of β-gal+ fibres counted on the total fibre number. Different muscles were analysed. Number of experimental animals: n =15 for Tg: TN-AP-CreERT2:R26R mice, black bars; n =5 for Tg:TN-AP-CreERT2:R26 NZG , red bars. Error bars represent standard deviation. ( h ) β-gal activity measurement on muscle homogenates. Standard curve was obtained by different dilutions of CMV-Cre-R26 and wt muscles. β-gal activity obtained 1 week after the last tamoxifen injection in TN-AP-CreERT2:R26R mice (representing labelling of the vessels) was subtracted from the obtained values. QUA, Quadriceps ; GAS, Gastrocnemius ; TRIC, Triceps ; PECT, Pectoralis ; DIAPH, Diaphragm; ABD, Abdominal ; BICF, Biceps femoris . Number of experimental animals: n =5. Error bars represent standard deviation. ( i – k ) Muscle sections of Tg:TN-AP-CreERT2:R26 NZG injected with tamoxifen at P6–P8 and killed 2 months later, stained with X-gal and Eosin. Arrows show β-gal+ nuclei inside skeletal muscle fibres; arrowhead shows β-gal+ nuclei of vessel-associated cells. Scale bar, 100 μm ( i ) or 20 μm ( j , k ). Full size image Next, we investigated whether AP+ cells might contribute to the satellite cell pool. To this end, muscles of Tg:TN-AP-CreERT2:R26R mice were collected at different time points after tamoxifen induction. No β-gal+/Pax7+ satellite cells were observed in vivo 3 days after the last tamoxifen injection; moreover, freshly isolated satellite cells did not express β-gal activity. However, 1 week after tamoxifen injection, few double-positive satellite cells were identified in vivo ( Fig. 4a ) (0.19% of the total Pax7+ cells in the TA and 2.5% in the Pectoralis ). At later stages, the percentage of double-positive Pax7+/β-gal+ satellite cells progressively increased in all muscles analysed, reaching, for example, 25% of total Pax7+ cells at 1 month after tamoxifen injection in the Pectoralis muscle ( Fig. 4b ). 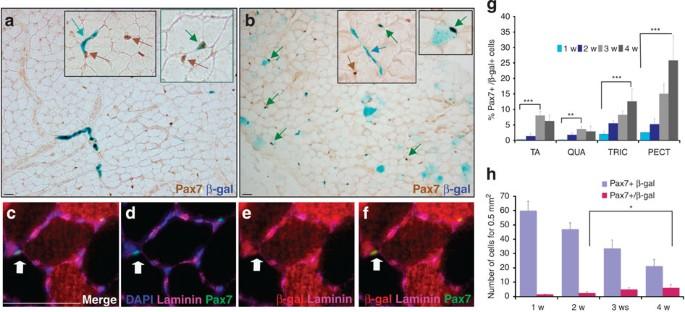Figure 4: Generation of satellite cells from AP+-derived cells during mouse growth. (a) Immunohistochemistry onTg:TN-AP-CreERT2:R26R Pectoralismuscle sections, 1 week after tamoxifen injection, stained for β-gal (blue) and anti-Pax7 (brown). The majority of Pax7+ cells are β-gal negative (brown arrows), whereas vessels are blue (blue arrows). Only few double-positive cells are detectable (green arrow). Insets show high magnification. (b) Immunohistochemistry onTg:TN-AP-CreERT2:R26R Pectoralismuscle sections 1 month after last tamoxifen injection stained for β-gal (blue) and Pax7 (brown). Several Pax7+/β-gal+ satellite cells were detected (green arrows) together with β-gal+ fibres. Insets show high magnification. (c–f)TAmuscle section ofTg:TN-AP-CreERT2:R26Rmouse, 2 months after tamoxifen injection. A Pax7+ (green) satellite cell also expresses β-gal (red) (arrows); the satellite cell is associated to a β-gal-negative fibre. Laminin is stained in magenta. Scale bar, 100 μm. (g) Pax7+/β-gal+ satellite cells counted on the total number of Pax7+ satellite cells, in different muscles and at different time points after tamoxifen induction: 1 week (pale blue), 2 weeks (dark blue), 3 weeks (pale grey), 4 weeks (dark grey). Number of experimental animals:n=5. Error bars indicate standard deviation. Results were assessed for statistical significance by Student'st-test (unpaired, two-tailed) and differences were considered statistically significant atP<0.05. Asterisks in the histogram indicate the differentPvalues: **P<0.01 and ***P<0.001. (h) Total number of satellite cells for microscopic field (~0.5 mm2) at different time points after tamoxifen induction inPectoralismuscle. Blue bars indicate the number of Pax7+/β-gal− satellite cells; red bars indicate the number of Pax7+/β-gal+ satellite cells. The total number of Pax7+ cells decreases with time, whereas the number of double-positive Pax7+/β-gal+ cells increases until 3 weeks after tamoxifen induction, remaining constant afterwards. Number of experimental animals:n=5. Error bars indicate standard deviation. Results were assessed for statistical significance by Student'st-test (unpaired, two-tailed) and differences were considered statistically significant atP<0.05. Asterisk in the histogram indicatesPvalue: *P<0.05. An example of Pax7+/β-gal+ satellite cells underneath the basal lamina of a β-gal-negative fibre is shown in Figure 4c–f . Quantifications of Pax7+/β-gal+ satellite cells detected with time are shown in Figure 4g . Although the total number of Pax7+ satellite cells decreases with time, the number of double-positive Pax7+/β-gal+ progressively increases, reaching a plateau at 3 weeks after tamoxifen induction; a detailed quantification for the Pectoralis muscle is shown in Figure 4h . Interestingly, we found a higher number of double-positive Pax7+/β-gal+ cells in the same muscles where we detected more β-gal+ fibres, suggesting that AP-derived cells contribute to skeletal muscle formation mainly by entering the satellite cell compartment, although direct fusion with developing muscle fibres may occur as well. Figure 4: Generation of satellite cells from AP+-derived cells during mouse growth. ( a ) Immunohistochemistry on Tg:TN-AP-CreERT2:R26R Pectoralis muscle sections, 1 week after tamoxifen injection, stained for β-gal (blue) and anti-Pax7 (brown). The majority of Pax7+ cells are β-gal negative (brown arrows), whereas vessels are blue (blue arrows). Only few double-positive cells are detectable (green arrow). Insets show high magnification. ( b ) Immunohistochemistry on Tg:TN-AP-CreERT2:R26R Pectoralis muscle sections 1 month after last tamoxifen injection stained for β-gal (blue) and Pax7 (brown). Several Pax7+/β-gal+ satellite cells were detected (green arrows) together with β-gal+ fibres. Insets show high magnification. ( c – f ) TA muscle section of Tg:TN-AP-CreERT2:R26R mouse, 2 months after tamoxifen injection. A Pax7+ (green) satellite cell also expresses β-gal (red) (arrows); the satellite cell is associated to a β-gal-negative fibre. Laminin is stained in magenta. Scale bar, 100 μm. ( g ) Pax7+/β-gal+ satellite cells counted on the total number of Pax7+ satellite cells, in different muscles and at different time points after tamoxifen induction: 1 week (pale blue), 2 weeks (dark blue), 3 weeks (pale grey), 4 weeks (dark grey). Number of experimental animals: n =5. Error bars indicate standard deviation. Results were assessed for statistical significance by Student's t -test (unpaired, two-tailed) and differences were considered statistically significant at P <0.05. Asterisks in the histogram indicate the different P values: ** P <0.01 and *** P <0.001. ( h ) Total number of satellite cells for microscopic field (~0.5 mm 2 ) at different time points after tamoxifen induction in Pectoralis muscle. Blue bars indicate the number of Pax7+/β-gal− satellite cells; red bars indicate the number of Pax7+/β-gal+ satellite cells. The total number of Pax7+ cells decreases with time, whereas the number of double-positive Pax7+/β-gal+ cells increases until 3 weeks after tamoxifen induction, remaining constant afterwards. Number of experimental animals: n =5. Error bars indicate standard deviation. Results were assessed for statistical significance by Student's t -test (unpaired, two-tailed) and differences were considered statistically significant at P <0.05. Asterisk in the histogram indicates P value: * P <0.05. Full size image Muscle regeneration enhances AP+ pericyte myogenesis Tg:TN-AP-CreERT2:R26R mice were treated with tamoxifen at P6–P8 and then injected with cardiotoxin in TA and Gastrocnemius muscles at P30; three weeks after injury all treated muscles showed a strong increase in the percentage of β-gal+ fibres in comparison with the contralateral, uninjured muscle ( Fig. 5a,b ). 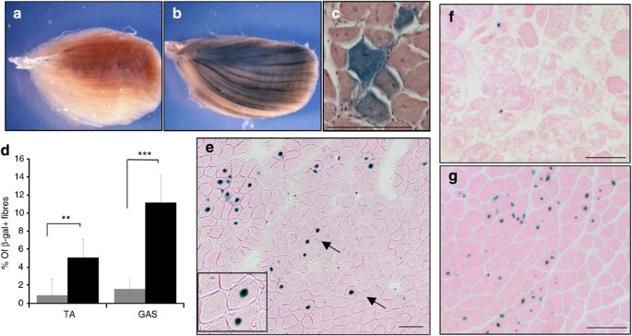Figure 5: AP+ pericytes contribution to skeletal muscle after acute injury. (a,b) Whole-mount X-Gal staining ofTg:TN-AP-CreERT2:R26Runtreated (a) or cardiotoxin-treated (b)TAmuscle showing a dramatic increase in the number of β-gal+, regenerated fibres. (c) Section of muscles shown in (b), stained for β-gal and H&E; β-gal+ centrally nucleated fibres are visible. (d) The percentage of β-gal+ fibres is increased from 0.9% in untreatedTAmuscle (grey histogram) to 5.07% in cardiotoxin-treatedTAmuscle (black histogram). InGastrocnemius(GAS), the percentage of β-gal+ fibres is increased from 1.6% in untreated leg (grey histogram) to 11.15% in cardiotoxin-treated (black histogram). Number of experimental animals:n=5; error bars indicate standard deviation. Results were assessed for statistical significance by Student'st-test (unpaired, two-tailed) and differences were considered statistically significant atP<0.05. Asterisks in the histogram indicate the differentPvalues: **P<0.01 and ***P<0.001. (e)TAsection ofTg:TN-AP-CreERT2:RNZGmice injected with tamoxifen at P6–P8, treated with cardiotoxin at 3 weeks and killed 3 weeks after damage. Many regenerating, centrally nucleated fibres are present (arrows); high magnification is shown in the inset. (f,g)TAsections ofTg:TN-AP-CreERT2:RNZGmice injected with two rounds of cardiotoxin and killed 24 h (f) or 3 weeks (g) after the second injury (details in the text). Scale bar, 100 μm. A section at high magnification, showing centrally located nuclei, typical of regenerating fibres, is shown in Figure 5c ; quantification is shown in Figure 5d . These experiments were confirmed with Tg:TN-AP-CreERT2:R26R line #3 and using Tg:TN-AP-CreERT2:R26 NZG mice ( Fig. 5e ). Figure 5: AP+ pericytes contribution to skeletal muscle after acute injury. ( a , b ) Whole-mount X-Gal staining of Tg:TN-AP-CreERT2:R26R untreated ( a ) or cardiotoxin-treated ( b ) TA muscle showing a dramatic increase in the number of β-gal+, regenerated fibres. ( c ) Section of muscles shown in ( b ), stained for β-gal and H&E; β-gal+ centrally nucleated fibres are visible. ( d ) The percentage of β-gal+ fibres is increased from 0.9% in untreated TA muscle (grey histogram) to 5.07% in cardiotoxin-treated TA muscle (black histogram). In Gastrocnemius (GAS), the percentage of β-gal+ fibres is increased from 1.6% in untreated leg (grey histogram) to 11.15% in cardiotoxin-treated (black histogram). Number of experimental animals: n =5; error bars indicate standard deviation. Results were assessed for statistical significance by Student's t -test (unpaired, two-tailed) and differences were considered statistically significant at P <0.05. Asterisks in the histogram indicate the different P values: ** P <0.01 and *** P <0.001. ( e ) TA section of Tg:TN-AP-CreERT2:R NZG mice injected with tamoxifen at P6–P8, treated with cardiotoxin at 3 weeks and killed 3 weeks after damage. Many regenerating, centrally nucleated fibres are present (arrows); high magnification is shown in the inset. ( f , g ) TA sections of Tg:TN-AP-CreERT2:R NZG mice injected with two rounds of cardiotoxin and killed 24 h ( f ) or 3 weeks ( g ) after the second injury (details in the text). Scale bar, 100 μm. Full size image To investigate whether AP+ pericyte-derived satellite cells were able to support a second round of regeneration, six Tg:TN-AP-CreERT2:R26 NZG mice at 1 month of age were injected with cardiotoxin in both TA , as described above. After three weeks, a second cardiotoxin injection (at the same dose) was performed in the right TA only. Mice killed 24 h after the second injection showed complete destruction of previously regenerated fibres ( Fig. 5f ), as compared with contralateral muscles that had received only one injection and appeared similar to what shown in Figure 5e . Mice killed after three extra weeks showed the presence of new β-gal+, centrally nucleated fibres ( Fig. 5g ). Muscular dystrophy also enhances AP+ pericyte myogenesis To test whether AP+ pericytes increase their contribution to skeletal muscle during the degeneration/regeneration cycles that characterize the progression of muscular dystrophy, Tg:TN-AP-CreERT2:R26R: α SG−/− dystrophic pups and their heterozygous littermates Tg:TN-AP-CreERT2:R26R: α SG+/− were injected with tamoxifen at P6–P8 and killed 2 months later. In dystrophic skeletal muscle, we observed a very high percentage of β-gal+ fibres, up to three times more than control mice ( Fig. 6a,b ). Skeletal muscle sections showed that the regenerated fibres robustly express β-gal ( Fig. 6c ; quantification in Fig. 6d ). 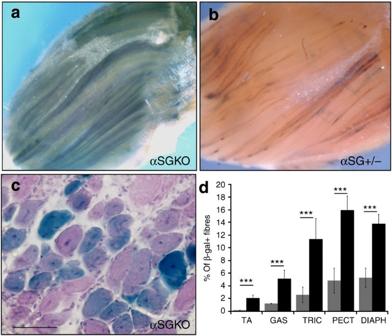Figure 6: AP+ pericytes contribution to skeletal muscle during chronic regeneration. (a,b)Tricepsmuscles ofTg:TN-AP-CreERT2:R26R:αSGKO(a) orTg:TN-AP-CreERT2:R26R:αSG+/−(b) mice, injected with tamoxifen at P6–P8, killed two months later and stained for β-gal activity. Many β-gal+ fibres can be detected in the dystrophic muscle. (c) Muscle sections ofTg:TN-AP-CreERT2:R26R:αSGKOshown in (a) stained for β-gal and H&E. Scale bar, 100 μm. (d) Percentage of β-gal+ fibres detected in the dystrophic muscles. Grey bars indicate αSG+/−background; black bars indicate αSGKObackground. Number of experimental animals:n=5; error bars indicate standard deviation. Results were assessed for statistical significance by Student'st-test (unpaired, two-tailed) and differences were considered statistically significant atP<0.05. Asterisks in the histogram indicate thePvalue: ***P<0.001. GAS,Gastrocnemius; TRIC,Triceps; PECT,Pectoralis; DIAPH, Diaphragm. Figure 6: AP+ pericytes contribution to skeletal muscle during chronic regeneration. ( a , b ) Triceps muscles of Tg:TN-AP-CreERT2:R26R: α SGKO ( a ) or Tg:TN-AP-CreERT2:R26R: α SG+/− ( b ) mice, injected with tamoxifen at P6–P8, killed two months later and stained for β-gal activity. Many β-gal+ fibres can be detected in the dystrophic muscle. ( c ) Muscle sections of Tg:TN-AP-CreERT2:R26R: α SGKO shown in ( a ) stained for β-gal and H&E. Scale bar, 100 μm. ( d ) Percentage of β-gal+ fibres detected in the dystrophic muscles. Grey bars indicate α SG+/− background; black bars indicate α SGKO background. Number of experimental animals: n =5; error bars indicate standard deviation. Results were assessed for statistical significance by Student's t -test (unpaired, two-tailed) and differences were considered statistically significant at P <0.05. Asterisks in the histogram indicate the P value: *** P <0.001. GAS, Gastrocnemius ; TRIC, Triceps ; PECT, Pectoralis ; DIAPH, Diaphragm. Full size image AP+ pericyte myogenesis is minimal in adult muscle Two- and three-month-old male Tg:TN-AP-CreERT2:R26R mice were treated intraperitoneally with tamoxifen for 3 consecutive days and, 1 week after tamoxifen injection, almost 70% of AP+ cells were β-gal+. β-gal expression always co-localized with Pecam+ or NG2+ vessel-associated cells ( Supplementary Fig. S3a,b ). Two months after tamoxifen injection, all muscles examined showed many β-gal+ vessels; in ~30% of treated mice, we detected very few β-gal+ fibres, only short fragments of which were labelled, suggesting focal contribution of few AP-derived cells during adult life ( Supplementary Fig. S3c ). Moreover, this minimal contribution did not significantly increase after cardiotoxin-induced regeneration (0.15±0.1 in control TA and 0.93±0.4 in cardiotoxin TA ; n =4) ( Supplementary Fig. S3e–h ; quantification in Supplementary Fig. S3d ). The contribution did not increase even when mice were injected with tamoxifen for 5 consecutive days. Endothelial cells do not contribute to postnatal myogenesis As AP is expressed in both pericytes and endothelial cells, we investigated whether one or both cell types contribute to skeletal muscle formation in vivo . Tg:VE-cadherin -( PAC ) CreERT2:R26R mice [13] were injected at P6–P8 with tamoxifen. Because VE-Cadherin is expressed only in endothelial cells [22] , we could selectively follow the fate of these cells. Three days after induction, 87±5% of total vessels were β-gal+ ( Fig. 7a ) and remained β-gal+ even in the mouse adult life ( Fig. 7b,c ), indicating a very efficient recombination in this transgenic mouse strain. Neither satellite cells nor myofibres were labelled 3 days or 1 week after tamoxifen injection ( Fig. 7d ) or, most importantly, 1 or 2 months after tamoxifen injection, in any of the muscles analysed ( Fig. 7e ). This was also the case after muscle regeneration induced by cardiotoxin injection ( Fig. 7f,g ). Taken together, these results indicate that in postnatal life, endothelial cells do not contribute to skeletal muscle growth or regeneration, nor to the satellite cell pool. 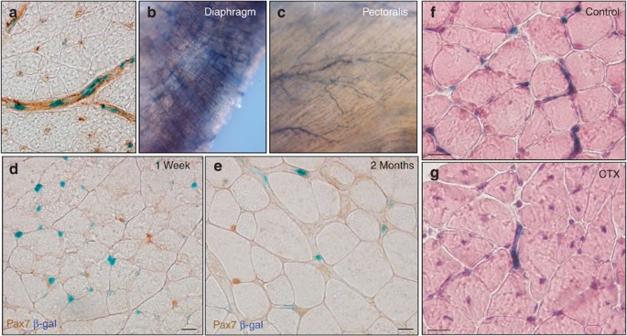Figure 7: Endothelial cells do not contribute to growing or regenerating muscle. (a)Ve-cadherin(PAC)-CreRT2:R26R Pectoralismuscle stained for β-gal (blue) and Pecam (brown) 3 days after tamoxifen injections (P6–P8). (b,c) Whole mount X-Gal staining ofVe-cadherin(PAC)-CreRT2:R26RDiaphragm (b) andPectoralis(c) 2 months after tamoxifen injections (P6–P8). β-gal+ vessels are clearly visible. (d,e)TAmuscle sections ofVe-cadherin(PAC)-CreERT2:R26Rmouse 1 week (d) and 2 months (e) after tamoxifen injection, stained for β-gal (blue) and anti-Pax7 (brown). No double-positive cells are present. (f,g)TAmuscle sections ofVe-cadherin(PAC)-CreERT2:R26Rmice 1 month after cardiotoxin injection (CTX) (g) and contralateral muscle (f), stained for β-gal and H&E. No β-gal+ fibres are detected. Scale bar, 20 μm. Figure 7: Endothelial cells do not contribute to growing or regenerating muscle. ( a ) Ve-cadherin ( PAC ) -CreRT2:R26R Pectoralis muscle stained for β-gal (blue) and Pecam (brown) 3 days after tamoxifen injections (P6–P8). ( b , c ) Whole mount X-Gal staining of Ve-cadherin ( PAC ) -CreRT2:R26R Diaphragm ( b ) and Pectoralis ( c ) 2 months after tamoxifen injections (P6–P8). β-gal+ vessels are clearly visible. ( d , e ) TA muscle sections of Ve-cadherin ( PAC ) -CreERT2:R26R mouse 1 week ( d ) and 2 months ( e ) after tamoxifen injection, stained for β-gal (blue) and anti-Pax7 (brown). No double-positive cells are present. ( f , g ) TA muscle sections of Ve-cadherin ( PAC ) -CreERT2:R26R mice 1 month after cardiotoxin injection (CTX) ( g ) and contralateral muscle ( f ), stained for β-gal and H&E. No β-gal+ fibres are detected. Scale bar, 20 μm. Full size image AP+ cells generate smooth or skeletal myogenic clones in vitro To confirm a possible progressive recruitment of AP+ cells into the satellite cell compartment, YFP+ cells, isolated from Tg:TN-AP-CreERT2:R26R-EYFP mice ( Fig. 8a ) at different time points (3 days, 1 week, 1 and 2 months) after tamoxifen injection (P6–P8), were stained for Pax7 ( Fig. 8c–e ; quantification Fig. 8b ). The percentage of double-positive Pax7+/YFP+ cells progressively increased during the first month of life from 0%, 3 days after tamoxifen injection, to 3.7±1.4% after 1 week, and 25.7±2.9% after 1 month, remaining at a similar level at 2 months (30.3±5.2%). One month after cardiotoxin muscle injury, tamoxifen-treated mice showed a similar percentage of YFP+ cells co-expressing Pax7 (29.5±5.4%) ( Fig. 8b ), suggesting that AP-derived satellite cells can self-renew and maintain a constant contribution to the satellite cell pool. These results were confirmed by quantitative RT–PCR for Pax7 and Myf5 ( Supplementary Fig. S4a ). Surprisingly, AP-derived satellite cells did not express Myf5 , suggesting that they may belong to the Pax7+/Myf5−, self-renewing satellite cell population [23] . 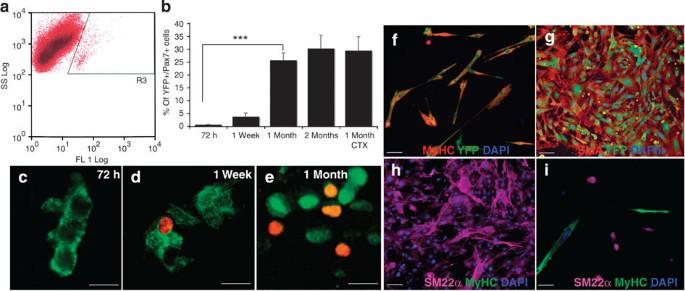Figure 8: Myogenic potential of isolated AP-derived YFP+ cells. (a) FACS analysis with a gate selected to sort YFP+ cells. (b) Relative frequency of double-positive YFP+/Pax7+ cells as % of the total YFP+ cells, obtained immediately after sorting, at different time points after tamoxifen induction and after cardiotoxin injection (CTX). Error bars indicate standard deviation. Results were assessed for statistical significance by Student'st-test (unpaired, two-tailed), and differences were considered statistically significant atP<0.05. Asterisks in the histogram indicate the differentPvalues: ***P<0.001. (c–e) Freshly isolated YFP+ cells were stained with anti-GFP antibody (green) and anti-Pax7 (red). Scale bar, 20 μm (f) Skeletal myogenic YFP+ clone, stained with anti-MyHC (red), anti-GFP (green) and DAPI (blue). (g) Smooth myogenic YFP+ clone, stained with anti-SMA (red), anti-GFP (green) and DAPI (blue). (h,i) Smooth myogenic (h) and mixed (i) YFP+ clones stained for anti-MyHC (green), anti-SM22α (magenta) and DAPI (blue). We counted 2 double-positive clones on a total number of 114 clones scored. Scale bars, 40 μm. Figure 8: Myogenic potential of isolated AP-derived YFP+ cells. ( a ) FACS analysis with a gate selected to sort YFP+ cells. ( b ) Relative frequency of double-positive YFP+/Pax7+ cells as % of the total YFP+ cells, obtained immediately after sorting, at different time points after tamoxifen induction and after cardiotoxin injection (CTX). Error bars indicate standard deviation. Results were assessed for statistical significance by Student's t -test (unpaired, two-tailed), and differences were considered statistically significant at P <0.05. Asterisks in the histogram indicate the different P values: *** P <0.001. ( c – e ) Freshly isolated YFP+ cells were stained with anti-GFP antibody (green) and anti-Pax7 (red). Scale bar, 20 μm ( f ) Skeletal myogenic YFP+ clone, stained with anti-MyHC (red), anti-GFP (green) and DAPI (blue). ( g ) Smooth myogenic YFP+ clone, stained with anti-SMA (red), anti-GFP (green) and DAPI (blue). ( h , i ) Smooth myogenic ( h ) and mixed ( i ) YFP+ clones stained for anti-MyHC (green), anti-SM22α (magenta) and DAPI (blue). We counted 2 double-positive clones on a total number of 114 clones scored. Scale bars, 40 μm. Full size image To test the skeletal myogenic potential of AP-expressing vascular progenitors, we analysed the ability of AP-derived cells to give rise to myogenic clones. YFP+ cells were isolated 1 week after tamoxifen induction (P6–P8) and plated at clonal density in 96 multiwells (1 cell per well). On average, 10% of plated cells gave rise to clones and 30% of these clones contained MyHC-expressing myocytes and myotubes ( Fig. 8f ), indicating that AP-Cre+, vessel-associated cells have a significant spontaneous myogenic potential after isolation. Most (>90%) of the remaining MyHC-negative clones expressed smooth muscle actin (SMA) ( Fig. 8g ), in agreement with their pericyte origin and smooth muscle fate. This was confirmed by staining with an antibody recognizing the cytoskeletal protein SM22α, a smooth muscle-specific marker [24] ( Fig. 8h ); very few clones (less than 1%) contained both MyHC+ and SM22α+ cells ( Fig. 8i ), indicating that very few AP+ cells maintain a double potency, once isolated and cloned in vitro . Freshly isolated YFP+ cells express pericyte and endothelial genes such as Tie2, (endothelial-specific receptor tyrosine kinase 2), VEGFR2 (vascular endothelial growth factor receptor 2), AnnexinV, SMA and PDGFRβ ( Supplementary Fig. S4b ) and, on in vitro culture, YFP+ cells maintain pericyte markers such as NG2, SMA and desmin ( Supplementary Fig. S4c–e ). To further investigate the myogenic differentiation process of AP-derived pericytes and its relation with muscles expressing Pax3 in vivo , we sorted YFP+ cells from forelimb muscles (whose satellite cells are known to express Pax3) and hindlimb muscles of Tg:TN-AP-CreERT2:R26R-EYFP mice, either 1 and 8 weeks after last tamoxifen injection. At different times in culture, we followed Pax7, Pax3 and Myf5 expression by immuno-fluorescence. A high percentage of YFP+ cells, sorted 1 week after last tamoxifen injection, was found to express Pax3; 60% of the total YFP+ cells from the forelimb, and 25% from hindlimb ( Supplementary Fig. 5a–c ). Pax3 expression rapidly decreases after 48 h in culture, when Myf5 expression first appears. Pax7 is never expressed in culture, indicating that the myogenic differentiation of AP-derived pericytes, in culture, is Pax7-independent ( Supplementary Fig. S5d–f ). On the other hand, the protein expression profile of YFP+ cells sorted from Tg:TN-AP-CreERT2:R26R-EYFP , 8 weeks after last tamoxifen injection, is different and comparable to the typical satellite cells profile. In fact, Pax7 is expressed in many cells (50%) until 72 h in culture and decreases thereafter with a concomitant increase of Myf5 expression ( Supplementary Fig. S5g–i ) At this stage Pax3 is present at a low frequency (below 10%) only in cells obtained from forelimb muscles. Quantification of myogenic gene expression in YFP+ cells during time in culture, is shown in Supplementary Figure S5j,k , respectively, 1 week or 8 weeks after tamoxifen injection. Direct quantitative comparisons between Pax3 and Pax7 is not possible since Pax3 is also expressed in some smooth muscle cells [25] whereas Pax7 is not. In both cases, YFP+ cells, obtained 1 week or 8 weeks after tamoxifen injection, begin to form myotubes after 5 days in culture. Each experiment was repeated three times with six mice each; polyclonal populations were analysed after 24 and 48 h in culture, whereas single cell-derived clones were analysed at later time points, when clones became clearly identifiable. Early post-natal myogenesis is predominantly effected by proliferation of juvenile satellite cells that contribute to the development of skeletal muscle by fusing with growing myofibres, and, to its regeneration, by repairing or replacing damaged or degenerated myofibres [26] . Nevertheless, in the last ten years, evidence has accumulated that other progenitors can contribute to skeletal muscle regeneration either by direct fusion or by entering the satellite cell pool [6] , [7] , [8] , [27] , [28] , [29] , [30] , [31] , [32] , [33] , [34] , [35] , [36] . When identified, the anatomical niche of these cells has been often associated with blood vessels (endothelial cells, pericytes and also haematopoietic cells). However, the embryonic origin of these unorthodox myogenic cells and their lineage relationship with satellite cells remain unknown. It was similarly unclear whether skeletal myogenesis is one possible developmental option of these non-myogenic progenitors, or whether it represents the artificial consequence of cell transplantation that, through occasional fusion with regenerating fibres, exposes the donor cell nucleus to the dominant effect of MyoD. In this work, we used Tg:TN-AP-CreERT2 mice to follow the fate of vessel-associated cells during postnatal muscle growth. AP is broadly expressed in many pre- and postnatal tissues, and in different cell types such as osteoblasts [37] , embryonic stem cells [38] , bone marrow stroma cells [39] , liver and kidney cells [40] , granulocytes [41] and B cells [42] ; however, in postnatal mouse striated muscles, AP is expressed only by vessel-associated cells, in both endothelial cells and pericytes, as previously reported [9] , [14] , [15] , [16] , and exhaustively confirmed in this work through a variety of histochemical and immunochemical methods. Most importantly, by using virtually all possible experimental approaches, we demonstrated that both AP and Cre expression are invariably absent in quiescent satellite cells, as well as in proliferating and differentiating myogenic cells in vitro or in vivo , even after cardiotoxin-induced damage. These preliminary results rule out the possibility of inappropriate lineage tracing, because of undetected expression in different cell types resident in skeletal muscle, and allowed us to investigate the fate of AP-derived vascular cells in growing postnatal skeletal muscle. A time course of reporter gene expression showed that, beside their expected contribution to the micro-vascular wall, pericytes, but not endothelial cells (as revealed by an endothelial-specific CreERT2 mouse), contribute to the growth of a minor but significant percentage of muscle fibres. Moreover, many AP-derived cells enter the satellite cell pool, with a relatively fast kinetics during the first month of postnatal life, suggesting that they also contribute to subsequent muscle regeneration. Indeed, conditions that trigger acute or chronic skeletal muscle regeneration, such as cardiotoxin injection or muscular dystrophy, increase dramatically AP+ cell contribution to skeletal myogenesis (up to five times in the area of acute regeneration and three times in dystrophic muscle). These results show that AP+ pericytes respond to pathological conditions, and, thus, they may serve as a tool for the cell therapy of dystrophic patients and justify the rationale for a clinical trial, with human AP+ pericytes, that is currently running in our Institution. We found the highest number of β-gal+ fibres and β-gal+ satellite cells in muscles where Pax3 is expressed postnatally, such as forelimb muscles and Diaphragm [43] . Furthermore, we observed that these AP+ vessel-associated cells express Pax3 in young animals (D.A., C.D. and C.G. ; unpublished data) and that YFP+ cells, isolated 1 week after tamoxifen injection, express Pax3, and not Pax7, in culture. On the other hand, we have clearly shown that, during mouse growth, AP-derived pericytes become real satellite cells and acquire Pax7+ expression in vivo , under the basal lamina and when isolated in vitro , two months after tamoxifen induction. It was previously demonstrated that during embryogenesis Pax3+ progenitors of the dermomyotome give rise not only to myogenic cells, but also to several other mesoderm cell types, including dermal fibroblasts, endothelial cells [44] , [45] and, notably, to pericytes and in the trunk and limbs smooth muscle of the dorsal aorta [25] . Thus, whereas all satellite cells appear to originate from somites [2] , the data presented here are not in contrast with this evidence, because other mesoderm progenitors, such as Pax3-expressing pericytes, also originate from somites. These progenitors may directly differentiate into skeletal muscle while expressing Pax3 (at least in vitro ), and this occurs more frequently in postnatal forelimb muscles where Pax3 is more abundant; alternatively, they may enter the satellite cells pool and activate Pax7 expression. AP+ cell contribution to skeletal muscle mainly occurs during the first month of postnatal growth and becomes sporadic in adult mice even in regenerating myofibres after cardiotoxin-induced muscle damage. Probably only during perinatal growth AP-derived pericytes can contribute to skeletal myogenesis and enter the satellite cells pool, in response to a major recruitment of myogenic cells to the maturing muscle fibres. Thus, it is conceivable that this contribution may be higher during prenatal development but, unfortunately, widespread expression of AP at this stage precludes this analysis. Very recently, three reports [46] , [47] , [48] showed that selective ablation of Pax7-expressing satellite cells during adult life permanently hampers subsequent attempts to regenerate skeletal muscles, leading to the conclusion that no other endogenous cell types may substitute for satellite cells. These results are not in contradiction with those reported here for the following reasons: the ablation of Pax7+ satellite cells was carried out in adult mice, at an age when the contribution of AP+ pericyets to muscle regeneration becomes negligible. It is also possible that satellite cells are required to induce other cell types to adopt a myogenic fate, as suggested by Sambasivan et al . [48] In conclusion, we have demonstrated that vascular pericytes, resident in skeletal muscle, are bi-potent (as confirmed by clonal analysis), as they contribute to both the smooth muscle layer of blood vessels and skeletal muscle fibre development, including the satellite cell pool, during unperturbed, postnatal growth of the mouse. It is still unknown how this choice is regulated in vivo , although it is plausible that signals emanating from neighbour muscle fibres or endothelium may direct the cells to a skeletal or to a smooth muscle fate, respectively. Mice generation and genotyping To generate Tg:TN-AP-CreERT2 mice the Cre recombinase fused with estrogen receptor (CreERT2) was cloned in a pGEM-T Easy Vector, between two fragments homologous to TN-AP gene in the starting coding region ATG upstream region. The construct was inserted into a bacterial artificial chromosome (BAC) 240 kbp clone (RP23 RP23-400F8 (Start: 137,302,861 and End: 137,529,460)) by homologous recombination in bacteria (spanning from 177 kbp upstream of the ATG, and covering most of the coding region). Molecular analysis demonstrated the correct insert of the construct into the BAC ( Supplementary Fig. S2b,c ). Digestion by BamHI shows the generation of an extra 2.8 kbp band and the absence of an 8 kbp band in the electroporated BAC compared with the unelectroporated one. Injection of the BAC into fertilized eggs generated a total of seven independent transgenic lines that were tested by crossing with the R26R reporter mouse [49] . Three lines were found to express beta-galactosidase and were used for subsequent experiments. Mice were kept heterozygous and genotyped by FW primer mapping on TN-AP sequence (FWTN-AP cgtctagatgagcctagggctggctggagcacag) and RW primer mapping on Cre sequence (RWCRE cagccaccagcttgcatga), generating a 1,400 bp band. Genotyping strategies of other mice, including Pax7−/− mutant mice [50] , Myf5 nlacZ/+ mice [19] , Ve-Cadherin -( PAC ) CreERT2 (ref. 12 ), TN-AP β geo/+ (ref. 16 ) have been published. To test our transgenic model, we used three different reporter mice: R26R [49] that express cytoplasmic β-gal; R26 NZG [21] that express nuclear β-gal and R26R-EYFP [51] that express cytoplasmic YFP. Control mice C57/BLJ6 from Jackson laboratory were used. All experiments were performed under internal regulations for animal care and handlings (IACUC 355). Both males and females were used for experiments and they were equally distributed between control and treated groups to avoid gender variations in muscle mass. Tamoxifen injection and cardiotoxin treatment Young animals were injected subcutaneously with 0.25 mg of tamoxifen, diluted in corn oil, (SIGMA T5648-1G) for 3 consecutive days at 6, 7 and 8 days after birth. Adult animals were treated for 3 consecutive days with 2 mg of tamoxifen by intraperitoneal injection. For the injury protocol, 25 μl of 100 μM cardiotoxin from Naja mossambica mossambica (SIGMA C9759) were injected directly into skeletal muscle. X-gal staining and immunohistochemistry Dissected muscles were fixed with paraformaldehyde (PFA) 4% and 0.25% glutaraldehyde for 30 min at 4 °C. After incubation in X-gal solution O/N at 37 °C, they were washed and dehydrated with increasing sucrose concentration (10–20 and 30%) for 20 min and then frozen within OCT. Eight μm cryostats sections were used for immunohistochemistry and stained with H&E when necessary. The endogenous peroxidases were blocked by H 2 O 2 30% in methanol for 30 min. The sections were then incubated with PBS 0.2% Triton 1% BSA for 30 min and with 10% donkey serum for 30 min. Primary antibody incubation was followed by secondary biotinilated antibody (Dako) and ABC kit (Vector Laboratories, PK-6100), enzymatic reaction with DAB (Sigma) was followed under microscope and stopped after the appropriated time. β-gal activity measurement Muscles were homogenized in buffer (0.25 M Tris pH 7.8, PMSF 1 mM), centrifuged at 15,000 g ×10 min at 4 °C, and extracted proteins were subsequently quantified by spectrophotometer with DC protein Assay (Biorad, 500-0114). 100 μg of protein were incubated with 500 μl of Z Buffer pH7 (60 mM Na 2 HPO 4 40 mM NaH 2 PO 4 10 mM KCl, 1 mM MgSO 4 , 50 mM b-Mercaptoethanol) and 100 μl of ONPG (o-nitrophenyl-b- D -galactoside) 4 mg ml −1 at 37 °C for 2.5 h. The reaction was blocked with 250 μl of Na 2 CO 3 and the level of β-gal activity was evaluated by reading the OD 420 at the spectrophotometer. To quantify the proportion of β-gal+ fibres in different muscles of Tg:TN-AP-CreERT2:R26R mice, we created a standard curve by mixing different proportions (from 0.1 to 50%) of muscle homogenates derived from wild-type and CMV-Cre-R26 mice. The proportion of β-gal activity only due to β-gal-positive fibres was calculated by subtracting the activity measured in muscles from Tg:TN-AP-CreERT2:R26R mice injected with tamoxifen and killed 1 week later, when the β-gal signal is present only in vessel-associated cells. Alkaline phosphatase reaction Different kits for AP enzymatic detection were used (see below) to exploit different reaction colours. Muscle sections were fixed with PFA 4% at 4 °C for 10 min and, after 3 washes, incubated with BCIP-NBT kit (Roche, 12296226 and 12329020) in an alkaline buffer (NaCl 100 mM, Tris 100 mM PH 9.5, MgCl 2 50 mM, Tween 0.1%) for 20 min in the dark, or with PermaRed/AP (Histo-Line laboratories, K049) for 20 min. Moreover, AP substrate kit from Vector (SK-5100) were used and visualized by confocal microscopy (Leica) at 456 nm, along with other immuofluorescent antibodies. Immunofluorescence and antibodies Frozen sections and cultured cells were fixed with PFA 4% at 4 °C for 10 min, washed 3× with Triton 0.2% BSA 1% in PBS, and incubated with the same buffer for 30 min, followed by 10% Donkey serum for 30 extra min. Primary antibody was incubated for 1 h at room temperature or O/N at 4 °C in the same buffer. Samples were washed 3 times and then incubated with secondary antibodies (Alexa Fluor 488-594-546 or 647, Invitrogen) for 1 h at RM, washed 3 times and then mounted and examined under epifluorescence or confocal Leica microscope. The immunofluorescence assay was carried out with the following antibodies: rabbit anti-β-galactosidase at 1:100 dilution (Chemicon, AB986), rabbit anti-β-gal at 1:1,000 (MPCappel 559762) and mouse anti-β-gal at 1:200 (Promega Z3783); rabbit anti-laminin at 1:300 (Sigma, L9393) or chicken anti-laminin at 1:500 (Abcam, Ab14055); anti- NG2 1:200 (Chemicon, AB5320) or donated from W. Stallcup, at 1:100; anti-Pecam at 1:2 (gift from Elisabetta Dejana); anti-Pax7 at 1:2 (DHSB); anti-smooth muscle actin at 1:200 (Sigma, A2547); anti-SM22α at 1:100 (Abcam); anti-MyHC at 1:2 (MF20 DHSB); anti-GFP 1:300 (Chemicon, AB3080); anti-Ki67 at 1:500 (Novo Castra, NCL-Ki67p), anti-PDGFRβ at 1:100 (from W. Stallcup), anti-AP at 1:100 (R&D); anti Pax3 at 1:2 (DHSB); anti MyoD at 1:100 (Dako). Cell sorting Dissected muscles were cut in small pieces and digested by collagenase D 0.1% (Roche, 1088866) and Trypsin 0.25% (Gibco, 15090-046) for 20 min at 37 °C, 2 or 3 cycles. After spin and filtration, the cells were collected in DMEM, 20%FBS, 2 mM EDTA, 20 mM HEPES or PBS 2% FBS, 2 mM EDTA when staining with SM/C2.6 (a gift from S. Takeda). Cell Sorting was carried out in MoFLo System (DAKO); sorted cells were either cloned in 96 wells or collected for RNA extraction. FACS analysis was performed by Canto (BD); data were analysed by FACSDiva software (BD). Sorted cells were cultured with DMEM (Sigma) 20%FBS on (low factor) Matrigel (BD, 354248) coated wells, in low (3%) oxygen incubator. RT–PCR and quantitative real-time PCR The RNA from sorted cells was collected by RNeasy mini (or micro) kit (Qiagen, 74104 and 74004) and converted into double-strand complementary DNA with the Superscript VILO cDNA systhesis kit (Invitrogen, 11754-050), according to the manufacturer's instructions. Real-time quantitative PCR analysis was carried out on cDNA from isolated cells by using an Mx3000P real-time PCR detection system (Stratagene). Each cDNA sample was amplified in duplicate by using the Express SYBR GreenER qPCR Supermix (Invitrogen, 11784-200). How to cite this article: Dellavalle, A. et al . Pericytes resident in postnatal skeletal muscle differentiate into muscle fibres and generate satellite cells. Nat. Commun. 2:499 doi: 10.1038/ncomms1508 (2011).